Nucleophilic aromatization of monoterpenes from isoprene under nickel/iodine cascade catalysis As a large number of organic compounds possessing two isoprene units, monoterpenes and monoterpenoids play important roles in pharmaceutical, cosmetic, agricultural, and food industries. In nature, monoterpenes are constructed from geranyl pyrophosphate (C10) via various transformations. Herein, the bulk C5 chemical—isoprene, is used for the creation of various monoterpenoids via a nucleophilic aromatization of monoterpenes under cascade catalysis of nickel and iodine. Drugs and oil mixtures from conifer and lemon can be convergently transformed to the desired monoterpenoid. Preliminary mechanistic studies are conducted to get insights about reaction pathway. Two types of cyclic monoterpenes can be respectively introduced onto two similar heterocycles via orthogonal C–H functionalization. And various hybrid terpenyl indoles are programmatically assembled from abundant C5 or C10 blocks. This work not only contributes a high chemo-, regio-, and redox-selective transformation of isoprene, but also provides a complementary approach for the creation of unnatural monoterpenoids. Owing to their unique pharmacological properties, such as antimicrobial, anti-inflammatory, antipruritic and analgesic activities [1] , [2] , [3] , [4] , monoterpenes and monoterpenoids have been widely applied in the clinical therapeutics and medicinal discovery. Besides, these compounds also play important roles in cosmetic, food and perfume industries [5] , [6] , [7] , [8] . In nature, isopentenyl pyrophosphate (IPP) and dimethylallyl pyrophosphate (DMAPP) are condensed to form the geranyl diphosphate (GPP) by geranyl pyrophosphate synthase (GPPase). Through a key intermediate (geranyl cation), cyclic or acyclic monoterpenes are synthesized from GPP under enzymatic catalysis [9] , [10] , [11] . Different monoterpenes could be further modified by other specific enzymes for the construction of various functionalized monoterpenoids (Fig. 1a ). Considering the importance of terpenoids, it has broad prospects and great value to develop selective synthesis of terpenoids from bulk chemicals by mimicking the biological process. Fig. 1: Catalytic construction of terpenoids. a Biosynthetic pathway for the construction and post-translational modification of C10 blocks; b Biomimetic nucleophilic reactions with isoprene under transition metal catalysis; c This work: Nucleophilic aromatization of monoterpenes from isoprene under nickel/iodine cascade catalysis. Full size image Given its characteristic structure and abundance, isoprene is undoubtedly the most cost-effective choice for biomimetic constructions of terpenoids. In terms of the synthesis of hemiterpenoids, various catalytic systems have been well developed under transition metal catalysis [12] , [13] , [14] , [15] , [16] , [17] , [18] , [19] , [20] , [21] , [22] , [23] , [24] , [25] , [26] , [27] , [28] , [29] , [30] , [31] , [32] , [33] , [34] , [35] . Besides, with the regulation of ligand, Beller, Finn, Réau, Navarro, Carbó and our group reported palladium catalyzed nucleophilic telomerization of isoprene to produce acyclic monoterpenoids [32] , [36] , [37] , [38] , [39] , [40] , [41] , [42] , [43] , [44] . Using nickel-aminophosphinite complexes, different dimers of isoprene mixed together with low yields in Mortreux’s work [45] . With the aid of N -heterocyclic carbene (NHC) ligands, we have recently demonstrated a selective heteroarylative cyclotelomerization of isoprene for the construction of cyclic monoterpenoids (Fig. 1b ) [35] , [46] . Given aromatic compounds play indispensable roles in a broad spectrum of industries, we wonder is it possible to develop a strategy for the creation of aromatic monoterpenoids with a distinctive selectivity. To realize this proposal, we had to address the following challenges: (1) Chemoselectivity. The existing literatures have demonstrated that the formation of hemiterpenoids (C5), acyclic monoterpenoids (C10) was more favorable over cyclic monoterpenoids (C10). (2) Regioselectivity. Owing to the existence of four electronically unbiased alkenyl carbons on isoprene, >90 cyclic nucleophilic dimerization isomers of isoprene could be yielded theoretically [23] . (3) Redoxselectivity. In order to realize the nucleophilic aromatization of cyclic monoterpene, up to 4 different hydrogen atoms have to be eliminated regioselectively. It poses high demands on the selectivity of the oxidation system and the compatibility of isoprene dimerization. By addressing these challenges, we herein demonstrate an efficient nucleophilic aromatization of monoterpenes from isoprene under nickel/iodine cascade catalysis (Fig. 1c ). Preliminary mechanistic studies were conducted to understand the cascade catalysis process. Meanwhile, convergent syntheses and orthogonal C–H functionalizations were presented to show the compatibility of this protocol. And various hybrid terpenyl indoles from the aromatic C10 products were created programmably. 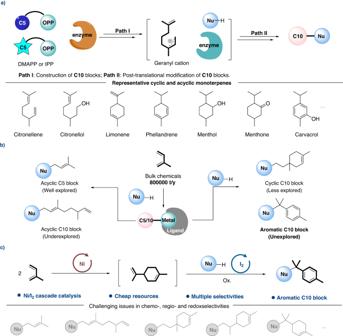Fig. 1: Catalytic construction of terpenoids. aBiosynthetic pathway for the construction and post-translational modification of C10 blocks;bBiomimetic nucleophilic reactions with isoprene under transition metal catalysis;cThis work: Nucleophilic aromatization of monoterpenes from isoprene under nickel/iodine cascade catalysis. Reaction optimization Unprotected indole 1a and isoprene 2a were chosen as model substrates for the investigation of nucleophilic aromatization under nickel/iodine cascade catalysis (Table 1 ). In the presence of K 2 S 2 O 8 , only prenylation products 3a , 4a (33% total yield) and diprenylated product 5a (20% yield) were detected using Ni(cod) 2 and I 2 as co-catalyst in one step procedure (entry 1). With the addition of IPr·HCl/NaO t Bu, the direct hydroarylation of isoprene was inhibited and no heteroarylative cyclotelomerization was observed (entry 2). When the reaction was carried out with two stepwise procedures in one-pot, aromatic C10 product 8a (28% yield) accompanied by trace of the other cyclic C10 products 6 and 7 was obtained when the temperature was increased from 80 to 100 o C (entries 3 and 4). Obvious impact on reactivities and selectivities was observed through the evaluation of ligands (entries 5–7). Bisphosphine ligand dppe only promoted the undesirable prenylation (entry 5). And the yield of targeted product 8a decreased significantly when using PCy 3 or less bulky IMes as ligand (entries 6 and 7 vs 4). The screening of solvents showed that nonpolar solvents such as toluene (48% yield of 8a ), n -hexane (51% yield of 8a ) for the first step brought better results (entries 8 and 9 vs 4). An obvious adverse effect on the formation of 8a when the solvent for the second step was changed from THF to 1,4-dioxane (entries 10 vs 4). Table 1 Optimization of reaction conditions a Full size table When DMSO was used instead of K 2 S 2 O 8 as oxidant [47] , reaction was completely unproductive (entry 11). The same result was also obtained as I 2 was replaced with NIS (entry 12). With the addition of catalytic amount of KI, the yield of 8a increased from 51% to 58% (entry 13). Besides, when using Na 2 S 2 O 8 instead of K 2 S 2 O 8 , the yield of desired product 8a could be further slightly improved (entry 14). Notably, acids showed to be effective additives to facilitate the reaction (entries 15 and 16), and (PhO) 2 PO 2 H emerged as the preferred additive for the formation of 8a (82% yield) in terms of reactivity and selectivity. Substrate scope With the optimized conditions in hand, we subsequently explored the generality of nucleophilic aromatization of monoterpenes from isoprene under nickel/iodine cascade catalysis (Fig. 2a ). Subjecting unsubstituted 1a to the standard conditions furnished aromatic C10-substituted indole 8a in 79% isolated yield. Methyl and fluorine on the phenyl ring, regardless of their positions, were all well-tolerated ( 8b, 8d, 8e, 8n and 8o ). In addition, indoles with either electron-donating (–OMe) or electron-withdrawing (–CN, –NO 2 , –CO 2 Me) substituents all reacted with isoprene 2a in good reactivities ( 8c and 8j - 8m , 51-94% yields). It is noteworthy that the common leaving groups such as –Cl, –Br, –I and –OTf, which could offer useful handles for further synthetic manipulations, were also compatible with the process to provide the corresponding products ( 8f – 8i ) in decent yields. Meanwhile, a scale-up experiment under the standard conditions was performed to afford the desired product 8a in 1.55 g with 78% yield. Fig. 2: Substrate scopes towards nucleophilic aromatization of isoprene. Conditions: Step I: 2a (1.2 mmol), Ni(cod) 2 /IPr·HCl (5.0 mol%), NaO t Bu (10 mol%), n -hexane (0.50 mL), 100 o C, 12 h; Step II: 1 (0.20 mmol), I 2 (20 mol%), KI/(PhO) 2 PO 2 H (10 mol%), Na 2 S 2 O 8 (2.0 equiv. ), THF (0.50 mL), 100 o C, 24 h. Isolated yields were given in all cases. Regio-selectivities were determined by 1 H NMR analysis. a 1a (8.0 mmol), 2a (48 mmol), n -hexane/THF (25 + 25 mL), 48 h for the second step; b 48 h for the second step; c 80 o C for the second step; d 1aa (0.10 mmol); e Filtration was required after the first step. Full size image For 3-substituted indole substrates, the C10 block could be introduced into the C 2 -site of indoles (Fig. 2b ). Various 3-Me indoles ( 1p - 1s ) were suitable substrates for the desired cross-coupling (58-81% yields). Notably, this transformation can be further extended to indole possessing ester-substituted alkyl group at C 3 position ( 1t ). For other nucleophiles, indazoles, benzotriazoles and pyrroles showed acceptable reactivities and selectivities (Fig. 2c ). With the enhancement of electron-withdrawing substituents, the reigoselectivities (N 1 or N 2 ) of indazoles decreased but the total yields were higher ( 8u – 8y ). In addition, when using benzotriazole as substrate, the regioselectivity was switched ( 8z , N 2 /N 1 = 3:1). Simple pyrrole 1aa could be modified by two C10 blocks simultaneously to give functionalized pyrrole 8aa . Besides, both 2-substituted and 2,3-disubstituted pyrroles ( 1bb and 1cc ) could be successfully applied in this transformation as well. In absence of the nickel, the targeted products could be observed using limonene instead of isoprene under I 2 catalysis. Control experiments further confirmed that I 2 and persulfate were indispensable for the process of nucleophilic aromatization (Please see Supplementary Tables 1 - 4 for details). Next, we sought out to assess the substrate scopes under the optimized condition (Fig. 3a ). The coupling of unprotected indole 1a and limonene 9a under oxidative condition gave the desired product 8a in 76% yield. Various indoles bearing –OMe, –F, –Br, and –I groups all reacted with limonene 9a in good reactivities ( 8c, 8d, 8g and 8h ). Notably, free hydroxyl substituted indole was also applicable ( 8dd ) and 5-CN or 6-CO 2 Me indole showed higher reactivities than the reaction from isoprene ( 8j and 8m ). In addition, 3-methyl indole and indazole also had good compatibility under this metal-free condition ( 8r and 8u ). Fig. 3: Substrate scopes towards nucleophilic aromatization of olefins. Conditions: 1 (0.20 mmol), 9 (0.30 mmol), I 2 (20 mol%), KI (10 mol%), K 2 S 2 O 8 (2.0 equiv. ), THF (0.50 mL), 100 o C, 12 h. Isolated yields were given in all cases. a 6 h; b 80 o C, 18 h; c 9 (0.40 mmol), K 2 S 2 O 8 (2.5 equiv. ), 24 h; d DMSO was used instead of K 2 S 2 O 8 , THF/MeNO 2 (0.50/0.50 mL), 24 h; e 18 h; f The proportion of each component was determined by the ratio of peak area of GC-FID and reactions (mixture of terprenes 54.5 mg) were conduted under the air atmosphere with 18 h; g 24 h; h A grain of limonene capsule; i 9 (0.25 mmol) without K 2 S 2 O 8 , 18 h. Full size image Other natural terpenoids were also applicable in this protocol (Fig. 3b ). Interestingly, an unusual cleavage of C–C bond occurred to give the product 8m when limonene 9a was replaced with carene, α-pinene or β-pinene ( 9c – 9e ). And an excellent result was obtained (91% yield of 8m ) when terpinolene, which has a tetrasubstituted C = C bond, was applied in the reaction ( 9f ). When K 2 S 2 O 8 was replaced with DMSO and a mixed solvent was used (THF/MeNO 2 = 1:1 v/v ), the couplings of carvone and dihydrocarvone ( 9g and 9h ) with indole exhibited good outcomes for hydroxyl product 8ee (71% and 43% yield, respectively). Besides, bisabolene, which is widely used in food flavors, could be converted into the product fitted with C15 block and an additional exocyclic C = C bond was formed simultaneously ( 8ff ). To illustrate the practical utility of this protocol, convergent synthesis was performed from the reaction of methyl indole-6-carboxylate 1m with mixture of olefins (Fig. 3c ). Good yield of 8m was obtained from the mixture of monoterpenes (limonene, carene, α-pinene, β-pinene and terpinolene, mixed in equal proportions). As an important industrial raw material extracted from coniferous plants, the turpentine mainly composed of α-pinene and β-pinene could afford the convergent product 8m in 63% yield. Commercially available limonene capsule was also attempted for the reaction and a satisfactory result (71% yield) was achieved. It’s worth noting that the peels of lemons and citrus, which are often thought as waste, contain high amounts of limonene and thus have the potential to be used as renewable materials. The distillate collected by a simple azeotropic distillation of lemon peel could be successfully applied in this transformation as well (75% yield). Meanwhile, the scope of aryl alkenes was investigated under the I 2 catalysis without the oxidants (Fig. 3d ). The reaction exhibited no obvious loss in both reactivities and selectivities when various (1,1-, 1-, and 1,2-)-substituted alkenes were subjected ( 8gg – 8jj ). In addition, this strategy can be further extended to 1,3-dienes and 4,3-hydroarylation products ( 8kk and 8ll ) could be obtained with high selectivities. These results also suggest that with the help of I 2 and oxidant, an oxidative aromatization of monoterpenes may take place before the nucleophilic addition during the aforementioned nucleophilic aromatization of monoterpenes. Mechanistic investigations In order to facilitate the exploration of mechanism, three sub-reactions (dimerization, oxidative aromatization, hydroarylation) were disassembled to study respectively. For cyclotelomerization, the kinetic experiment was carried out to interpret the process of generation of isoprene dimers under nickel catalysis (Fig. 4a ). The reaction steadily produced two [4 + 2] cycloaddition products 9a and 9b at the early stage. And quantitative conversion of isoprene was reached after five hours. Notably, no other cyclic or acyclic isomers were observed during this process. For aromatization, three isomerization products ( 10a, 10b and 9f ) and two aromatization products ( 11a and 12a ) were detected during the reaction of limonene 9a under I 2 catalysis (Fig. 4b ). At the beginning, limonene 9a was rapidly consumed to form the aforementioned products. The yield of 9f was higher than that of the other two isomers ( 10a and 10b ) and they all stayed at a low concentration with the consumption of limonene 9a . Meanwhile, two aromatization products ( 11a and 12a ) kept increasing until limonene 9a vanished. These results suggest that terpinolene 9f is probably the intermediate for the formation of aromatic products 11a and 12a through oxidation. Similar studies were conducted to figure out the mechanism when other monoterpenes (carene 9c , α-pinene 9d or β-pinene 9e ) replaced limonene 9a as substrates (Please see Supplementary Figs. 4 – 6 for details). Fig. 4: Mechanistic studies and proposed mechanism. a Kinetics experiment for the dimerization of isoprene 2a ; b Kinetics experiment for the aromatization of limonene 9a ; c Kinetics experiment for the coupling of 1a with 9a ; d Control experiments; e Proposed mechanism. Full size image For hydroarylation, the generation trend of these four products ( 10a, 10b, 9f and 11a ) is consistent with the process of aromatization, but 12a maintained at a lower concentration until the target product 8a no longer increased (Fig. 4c ). This indicates that aromatization product 12a may be the active intermediate. And the formation rate of 12a is slower in absence of KI (Please see Supplementary Fig. 10 for details). In contrast to the continuous increase of 8a , undesirable product 6 was produced only at the beginning of the reaction and then remained unchanged nearly. These results indicate the aromatization of cyclic monoterpene occurs before the hydroarylation. When 1,3-dideuterated indole was treated under the standard condition (Please see Supporting Information for details), both indole ring and aromatic C10 moiety were deuterated partially. The deuterium rate at C 2 of indole (23% D) was obviously higher than that at other sites, which indicates that C 2 of indole is more reactive under this protocol. Therefore, when active C 3 position of indole was substituted, the C10 block was easily introduced onto the C 2 site of indole. Furthermore, the KIE experiment (k H /k D = 1.23, see Supplementary Fig. 8 for details) suggests that the hydroarylation is probably not the rate-determining step. Additional control experiments were carried out to further elucidate the roles of potential intermediates (Fig. 4d ). When the reactions were conducted with substrates only bearing endocyclic double bonds, the side-products 6 rather than the desired product 8a were generated preferentially (Fig. 4d , entries 1 and 2). In comparison, olefin 9f which having exocyclic double bond was more inclined to form the target product 8a (Fig. 4d , entry 3). These results indicate that the double bond located at the isopropyl unit is the guarantee for the selective formation of 8a . In addition, triene 13a could also be transformed into 8a with 21% yield under the standard condition. Using HI (20 mol%) instead of the combo of I 2 , KI and K 2 S 2 O 8 , a higher yield of product 8a could be obtained from p -cymenene 12a through a Friedel-Crafts type reaction. Besides, when the mixture of 6 and 8a was added instead of indole and olefin into the reaction, no conversion of 6 into 8a was observed (Fig. 4d , entry 6). It ruled out the possibility that hydroarylation occurs before oxidative aromatization of monoterpenoid. On the basis of the above observations, a plausible mechanism was proposed for the nucleophilic aromatization of monoterpenes from isoprene via nickel and iodine catalysis (Fig. 4e ). For the isoprene 2a dimerization process, active Ni(0) species A which is formed in situ from Ni(cod) 2 , IPr·HCl and NaO t Bu firstly coordinates with one molecule isoprene 2a to generate the complex B . Subsequently, Ni complex B undergoes oxidative cyclometallation to give a five-membered nickelacycle C . Through the coordination with another isoprene 2a , complex D proceeds with a migratory insertion to furnish a seven-membered nickelacycle F via a transition state E . With the formation of new C–C bond, reductive elimination of Ni(II) species F yields the limonene 9a and active Ni(0) species A . There are two possible paths for nucleophilic aromatization (Fig. 4e , right) [48] , [49] , [50] . For path I, iodonium species G is initially obtained from limonene 9a with the help of I 2 . Through a nucleophilic attack by iodide, vicinal diiodide compound H is generated, which gives the intermediate 13a smoothly by an elimination of H–I. A subsequent 1,4-addition yields a skipped diiodide species J . And olefin 12a is formed from species J via double elimination of H–I. Finally, with the aid of the early released H–I, carbonium ion intermediate L is generated and reacts with nucleophile successfully to yield target product 8 . The required I 2 is regenerated from the oxidation of H–I by persulfate. For path II, an alkenyl isomerization 9a occurs to give more thermodynamic stable diene 9f . Through repeat processes of di-iodination/HI elimination ( 9f-K/K’−12a ), olefin 12a is then generated as the intermediate for the formation of desired product 8 . Inspired by parallel kinetic resolution, we envisioned whether it would be possible to develop a parallel transformation of these two regioisomers ( 9a and 9b ) of monoterpene with different nucleophiles in one same pot. As two important but similar heterocycles, benzofuran and indole were chosen as competitors for this proposal. Impressively, an orthogonal C–H monoterpenation of benzofuran and indole occurred smoothly to give product 15a and 8f in a chemo-, regio-, and redoxselective fashion. This orthogonal C–H functionalizations also showed good substrate generality (Fig. 5a ). Benzofurans bearing electron-donating (-OMe) and -withdrawing (-CO 2 Me) groups all underwent the desired cross-coupling smoothly ( 15b and 15c ). It should be noted that the borate group, which could be easily further modified, was well compatible under the current conditions ( 15d ). The phenyl group on different sites of phenyl ring had no significant impact on the reactions ( 15e vs 15f ). Fig. 5: Synthetic applications. a Orthogonal C–H functionalizations; b Concise and programmable construction of hybrid terpenyl indoles. Full size image Transformations The hybrid terpenyl indoles could be used as key building blocks in the total synthesis of a series of natural products. Thus, concise and divergent constructions of various hybrid terpenyl indoles have been demonstrated (Fig. 5b ). Treatment of 8a with a mixture of prenyl bromide and NaH successfully introduced linear C5 block onto the N atom of indole with high efficiency ( 16a ). Under palladium catalysis, reverse N-prenylation occurred to furnish the corresponding product 16b from 8a and 2-methyl-2-butene [51] . Through the strategy of dearomatization−rearomatization, N-cyclopentylindole 16c was formed with 57% yield in one step [52] . When using prenyl borates as C5 block, Pd-catalyzed Suzuki reaction underwent smoothly to deliver 5-prenyl indole 16d in 72% yield [53] . Furthermore, with the help of bases and additives, the linear and cyclic C10 blocks could be introduced into the N atom of indoles ( 16e vs 16f ) respectively [54] . For the another side of the indole ring, diaryl C10 product 16g could be accessed by a nickel catalyzed carbonyl-Heck reaction from cuminaldehyde and 8i [55] . Through a traditional Heck reaction, linear C10 compound 16h substituted at 5-position of indole was finally obtained in 82% yield [56] . In summary, a bioinspired nucleophilic aromatization of monoterpenes from isoprene has been developed under the cascade catalysis of nickel and iodine. Various nucleophiles such as indoles, indazoles, benzotriazole and pyrroles were suitable for this protocol. A series of natural terpenes were transformed to aromatic C10 or C15 blocks successfully by I 2 catalysis. Based on the good tolerance of different monoterpenes, convergent synthesis strategy was implemented smoothly by using drugs and plant extracts. Meanwhile, preliminary mechanistic studies provided evidence for possible catalytic pathways. Firstly, through the regulation of IPr ligand, the cyclodimerization of isoprene proceeds under Ni catalysis. Then, In the presence of K 2 S 2 O 8 , a highly selective nucleophilic addition occurs quickly following the oxidative aromatization of limonene under I 2 catalysis. An orthogonal C–H functionalization of two regioisomers of monoterpene with different nucleophiles was realized in one same pot. Moreover, various hybrid terpenyl indoles were programmatically assembled to illustrate the practical utility of this protocol. Further studies and application on transformations of isoprene are underway in our laboratory. General procedure for Ni/I 2 catalyzed nucleophilic aromatization from isoprene Step I: In a glove box, a sealed tube was charged with Ni(cod) 2 (0.01 mmol, 5.0 mol%), IPr·HCl (0.01 mmol, 5.0 mol%), NaO t Bu (0.02 mmol, 10 mol%), isoprene 2a (1.2 mmol), n -hexane (0.50 mL) at room temperature. The reaction tube was sealed with a Teflon screw cap and removed from the glove box. Then, the reaction mixture was stirred at 100 °C for 12 hours. Step II: As the reaction mixture was cooled to room temperature, (PhO) 2 PO 2 H (0.02 mmol, 10 mol%) was added to the reaction tube and stirred for 5 minutes. Then KI (0.02 mmol, 10 mol%), K 2 S 2 O 8 (0.40 mmol, 2.0 equiv. ), nucleophile 1 (0.20 mmol), I 2 (0.04 mmol, 20 mol%) and THF (0.50 mL) were added into the reaction mixture and stirred at 100 °C for additional 24 h. Direct purification by column chromatography on silica gel using petroleum ether and ethyl acetate afforded the corresponding product 8 . General procedure for I 2 catalyzed nucleophilic aromatization from terpenes In a glove box, a sealed tube was charged with KI (0.02 mmol, 10 mol%), K 2 S 2 O 8 (0.40 mmol, 2.0 equiv. ), nucleophile 1 (0.20 mmol), I 2 (0.04 mmol, 20 mol%), 9 (0.30 mmol) and THF (0.50 mL) at room temperature. The reaction tube was sealed with a Teflon screw cap and removed from the glove box. Then, the reaction mixture was stirred at 100 °C for 12 h. Direct purification by column chromatography on silica gel using petroleum ether and ethyl acetate afforded the corresponding product 8 . General procedure for I 2 catalyzed hydroarylation of olefins In a glove box, a sealed tube was charged with KI (0.02 mmol, 10 mol%), indole 1a (0.20 mmol), I 2 (0.04 mmol, 20 mol%), 9 (0.25 mmol) and THF (0.50 mL) at room temperature. The reaction tube was sealed with a Teflon screw cap and removed from the glove box. Then, the reaction mixture was stirred at 100 °C for 18 h. Direct purification by column chromatography on silica gel using petroleum ether and ethyl acetate afforded the corresponding product 8 . General procedure for Orthogonal C–H functionalizations Step I: In a glove box, a sealed tube was charged with Ni(cod) 2 (0.01 mmol, 5.0 mol%), IPr·HCl (0.01 mmol, 5.0 mol%), NaO t Bu (0.02 mmol, 10 mol%), benzofuran 14 (0.20 mmol), isoprene 2a (1.2 mmol), n -hexane (0.50 mL) at room temperature. 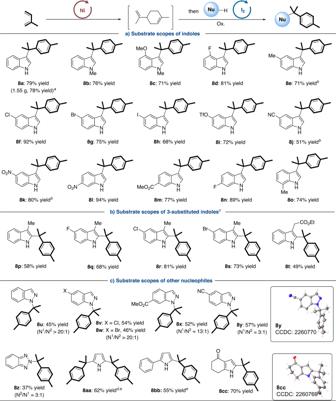Fig. 2: Substrate scopes towards nucleophilic aromatization of isoprene. Conditions: Step I:2a(1.2 mmol), Ni(cod)2/IPr·HCl (5.0 mol%), NaOtBu (10 mol%),n-hexane (0.50 mL), 100oC, 12 h; Step II:1(0.20 mmol), I2(20 mol%), KI/(PhO)2PO2H (10 mol%), Na2S2O8(2.0 equiv.), THF (0.50 mL), 100oC, 24 h. Isolated yields were given in all cases. Regio-selectivities were determined by1H NMR analysis.a1a(8.0 mmol),2a(48 mmol),n-hexane/THF (25 + 25 mL), 48 h for the second step;b48 h for the second step;c80oC for the second step;d1aa(0.10 mmol);eFiltration was required after the first step. The reaction tube was sealed with a Teflon screw cap and removed from the glove box. Then, the reaction mixture was stirred at 120 °C for 18 h. Step II: As the reaction mixture was cooled to room temperature, (PhO) 2 PO 2 H (0.02 mmol, 10 mol%) was added to the reaction tube and stirred for 5 min. Then, KI (0.02 mmol, 10 mol%), K 2 S 2 O 8 (0.40 mmol, 2.0 equiv. 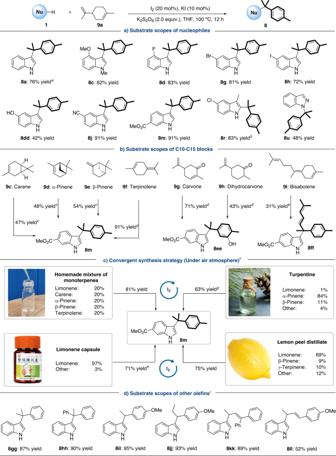Fig. 3: Substrate scopes towards nucleophilic aromatization of olefins. Conditions:1(0.20 mmol),9(0.30 mmol), I2(20 mol%), KI (10 mol%), K2S2O8(2.0 equiv.), THF (0.50 mL), 100oC, 12 h. Isolated yields were given in all cases.a6 h;b80oC, 18 h;c9(0.40 mmol), K2S2O8(2.5 equiv.), 24 h;dDMSO was used instead of K2S2O8, THF/MeNO2(0.50/0.50 mL), 24 h;e18 h;fThe proportion of each component was determined by the ratio of peak area of GC-FID and reactions (mixture of terprenes 54.5 mg) were conduted under the air atmosphere with 18 h;g24 h;hA grain of limonene capsule;i9(0.25 mmol) without K2S2O8, 18 h. 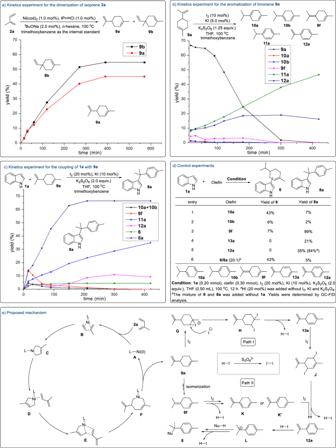Fig. 4: Mechanistic studies and proposed mechanism. aKinetics experiment for the dimerization of isoprene2a;bKinetics experiment for the aromatization of limonene9a;cKinetics experiment for the coupling of1awith9a;dControl experiments;eProposed mechanism. 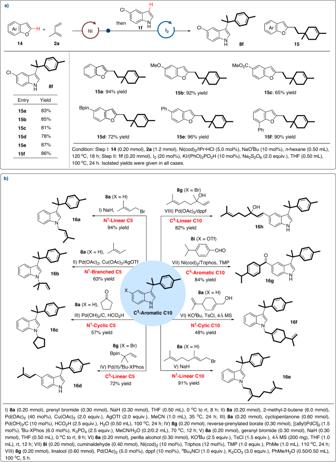Fig. 5: Synthetic applications. aOrthogonal C–H functionalizations;bConcise and programmable construction of hybrid terpenyl indoles. ), indole 1f (0.20 mmol), I 2 (0.04 mmol, 20 mol%) and THF (0.50 mL) were added into the reaction mixture and stirred at 100 °C for additional 24 h. Direct purification by column chromatography on silica gel using petroleum ether and ethyl acetate afforded the corresponding products 8f and 15 .